A disulphide-linked heterodimer of TWIK-1 and TREK-1 mediates passive conductance in astrocytes TWIK-1 is a member of the two-pore domain K + (K2P) channel family that plays an essential part in the regulation of resting membrane potential and cellular excitability. The physiological role of TWIK-1 has remained enigmatic because functional expression of TWIK-1 channels is elusive. Here we report that native TWIK-1 forms a functional channel at the plasma membrane of astrocytes. A search for TWIK-1-binding proteins led to the identification of TREK-1, another member of the K2P family. The TWIK-1/TREK-1 heterodimeric channel is formed via a disulphide bridge between residue C69 in TWIK-1 and C93 in TREK-1. Gene silencing demonstrates that surface expression of TWIK-1 and TREK-1 are interdependent. TWIK-1/TREK-1 heterodimers mediate astrocytic passive conductance and cannabinoid-induced glutamate release from astrocytes. Our study sheds new light on the diversity of K2P channels. The importance of K + currents for cellular excitability has been appreciated since the 1940, s, the era in which the principal concepts of electrophysiology were developed [1] . However, the molecular entities responsible for cellular K + currents have only recently been revealed. Two-pore domain K + (K2P) channels, the ‘leak channels’, are the last K + channel family to be discovered. They are major contributors to background K + conductance and they stabilize resting membrane potential as well as cellular excitability [2] . The first member of this family, K2P1 (TWIK-1; tandem of pore domains in a weak inward rectifying K + channel), was cloned from a human kidney cDNA library [3] , followed by the cloning of other members of this family, to finally reveal 15 mammalian isoforms of this channel. The K2P channel family are functional in adrenal gland development, thermal and mechanical nociception and show sensitivity to volatile anesthetics [2] . Although TWIK-1 was the first member of the K2P family to be cloned, TWIK-1 has long been considered to be non-functional. The electrophysiological properties and functional significance of TWIK-1 have remained enigmatic, due to the low or non-existent functional expression of TWIK-1 in heterologous expression systems. However, in endogenous systems, expression of TWIK-1 has been documented in various tissues, including the brain, heart and kidney [3] . Mice deficient in TWIK-1 show defects in phosphate transport in the proximal tubule and water transport in the medullary collecting duct of kidney, as well as deviations in the resting membrane potential of pancreatic β cells [4] , [5] . In addition, it has been recently reported that TWIK-1 conducts inward leak Na + currents during pathological hypokalaemia in cardiomyocytes [6] . These observations strongly suggest important physiological roles for TWIK-1 channels and imply the existence of control mechanisms for tight regulation of its functional expression. However, such possible roles remain hypothetical until actual K + currents carried by TWIK-1 are fully understood. There have been two distinct hypotheses that attempt to explain the low functional expression of TWIK-1. The first is that a special post-translational modification, called sumoylation, silences plasma membrane TWIK-1 channels [7] . This proposal was challenged by reports that TWIK-1 channels are not sumoylated [8] . The second is that TWIK-1 channels are silenced by constitutive endocytosis and intracellular sequestration [9] . However, neither hypothesis addresses the important question of how TWIK-1 actually functions as an ion channel and the role TWIK-1 plays, if any, in native systems. In contrast, a well-characterized K2P channel, TREK-1 (TWIK-related K + channel) was originally described as an outwardly rectifying K + channel [10] . Subsequent studies demonstrated that TREK-1 activity is regulated by multiple signals, such as polyunsaturated fatty acids, phospholipids, by stretch, and by intracellular acidification [11] , [12] , [13] , [14] , [15] . TREK-1 activity is also modulated by a host of G protein-coupled receptors (GPCRs) linked to G αs or G αq [16] , [17] . TREK-1 is highly expressed in neurons in many brain regions, including prefrontal cortex, hippocampus and hypothalamus [10] , [18] , [19] . In addition, we have recently shown that TREK-1 is also expressed in astrocytes within the brain and mediates rapid release of the gliotransmitter glutamate upon activation of GPCRs such as the cannabinoid receptor 1 (CB1), due to direct binding of G βγ to the N terminus of TREK-1 (ref. 20 ). Astrocytes have been reported to express TWIK-1 along with TREK-1 (ref. 21 ), but the relationship between these two channels has not yet been elucidated. Astrocytes have an unusually leaky membrane and extremely low membrane resistance. This property, termed passive conductance, typically exhibits a linear current–voltage relationship, which implies predominant expression of K + channels that differ from conventional voltage-gated or leak K + channels. Recently, the passive conductance of astrocytes has alluded to an independent contribution of TREK-1 and TWIK-1 (ref. 21 ), from a comparison made between biophysical and pharmacological properties of the passive conductance in astrocytes and of currents mediated by either a cloned TWIK-1 mutant (TWIK-1·K274E) or cloned TREK-1 channels in heterologous expression systems. However, the way in which native TWIK-1 contributes to the astrocytic passive conductance still remains to be determined. In the present study, we reveal native TWIK-1 currents in astrocytes and demonstrate that expression of functional TWIK-1 requires heterodimerization with TREK-1. We provide evidence to show that the TWIK-1/TREK-1 heterodimer mediates the K + current responsible for most of the background passive conductance in astrocytes and that it is also involved in CB1-induced fast glutamate release from these cells. TWIK-1 is a functional channel in astrocytes Although protein expression or mRNA of TWIK-1 has recently been reported in hippocampal astrocytes [21] , [22] , functional expression of native TWIK-1 protein has not been observed. To determine the subcellular localization of TWIK-1 in cultured hippocampal astrocytes, we performed immunocytochemistry with an anti-TWIK-1 antibody in astrocytes that overexpressed the plasma membrane marker, DsRed-Mem. Native TWIK-1 channels were highly localized at the plasma membrane of astrocytes, as evidenced by a yellow colour in the overlay or extracted co-localization images ( Fig. 1a ). This was strikingly different from the significantly lower surface expression and lack of TWIK-1-mediated currents in COS-7 cells having a heterologous expression of TWIK-1 ( Supplementary Fig. 1a,b ). A significantly higher expression of TWIK-1 at the plasma membrane of astrocytes was indicated by a higher value of Pearson’s correlation coefficient compared with that measured in COS-7 cells ( Fig. 1a ). Surface expression of TWIK-1 at the plasma membrane raised the possibility that TWIK-1 might act as a functional channel in astrocytes. To test this possibility, we first examined the effect of knocking down native TWIK-1 on the background conductance in astrocytes. For this purpose we developed a TWIK-1-specific short hairpin-forming interference RNA (shRNA) and an shRNA-insensitive form of mouse TWIK-1 (TWIK-1 insens WT: Supplementary Fig. 1c ). Individual cultured astrocytes showed a current–voltage ( I – V ) relationship with a complex shape, consisting of both outwardly rectifying outward current and weakly inwardly rectifying inward current ( Fig. 1b , black trace). TWIK-1 shRNA treatment significantly reduced both the outward and inward currents of astrocytes ( Fig. 1b,c ) and showed a positive shift in reversal potential from −79±2 mV to −52±4.7 mV ( Fig. 1d ), while the control scrambled shRNA (Sc shRNA) did not affect the I – V relationship or reversal potential ( Fig. 1b,d ). These effects of TWIK-1 shRNA were fully rescued by co-transfection of TWIK-1 shRNA with TWIK-1 insens WT ( Fig. 1b–d ). However, introducing a pore mutation at position 119, from glycine to glutamate (TWIK-1 insens G119E), failed to rescue the background conductance and reversal potential ( Fig. 1b–d ), indicating that it is the flow of K + through the pore of TWIK-1 that is responsible for the background conductance and resting membrane potential in astrocytes. The surface expression of TWIK-1 insens G119E in astrocytes was confirmed and compared with that of wild-type TWIK-1 by surface biotinylation ( Supplementary Fig. 1d ). Taken together, these results indicate that TWIK-1 forms a functional K + channel in cultured astrocytes. 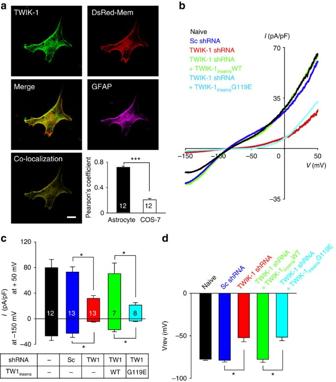Figure 1: TWIK-1 is a functional channel in astrocytes. (a) Plasma membrane localization of TWIK-1 in astrocytes. Astrocytes transfected with DsRed-Mem vector, as a specific marker for plasma membrane, were labelled with antibodies against TWIK-1 and GFAP. Representative images are shown in the top panels. Scale bar, 20 μm. Pearson’s correlation coefficient denoting covariance of fluorescence signals was calculated using Nikon software. The Pearson’s correlation coefficient for TWIK-1 and DsRed-Mem in astrocytes was significantly greater than values obtained in COS-7 cells. Number on each bar indicatesnfor each condition. All values are mean±s.e.m.P-values were obtained with Student’st-test. ***P<0.001. (b) Representative trace of naive (black), Sc shRNA (blue), TWIK-1 shRNA (red), TWIK-1 shRNA-insensitive (green) or TWIK-1 shRNA-insensitive pore mutant (G119E, cyan)-transfected astrocytes. The voltage ramp-induced whole-cell current traces recorded from each cell. (c) Summary bar graph of TWIK-1 shRNA (TW1 shRNA), TWIK-1 rescue (TW1insensWT) or TWIK-1 pore mutant (TW1insensG119E) rescue currents plotted at −150 mV and +50 mV. Number on each bar indicatesnfor each condition. All values are mean±s.e.m. (d) Reversal potential (Vrev) of astrocytes in the TW1 shRNA-transfected and TW1insensWT-transfected or TW1insensG119E-transfected cells. Number on each bar indicates n for each condition. All values are mean±s.e.m.P-values were obtained with Student’st-test. *P<0.05. Figure 1: TWIK-1 is a functional channel in astrocytes. ( a ) Plasma membrane localization of TWIK-1 in astrocytes. Astrocytes transfected with DsRed-Mem vector, as a specific marker for plasma membrane, were labelled with antibodies against TWIK-1 and GFAP. Representative images are shown in the top panels. Scale bar, 20 μm. Pearson’s correlation coefficient denoting covariance of fluorescence signals was calculated using Nikon software. The Pearson’s correlation coefficient for TWIK-1 and DsRed-Mem in astrocytes was significantly greater than values obtained in COS-7 cells. Number on each bar indicates n for each condition. All values are mean±s.e.m. P -values were obtained with Student’s t -test. *** P <0.001. ( b ) Representative trace of naive (black), Sc shRNA (blue), TWIK-1 shRNA (red), TWIK-1 shRNA-insensitive (green) or TWIK-1 shRNA-insensitive pore mutant (G119E, cyan)-transfected astrocytes. The voltage ramp-induced whole-cell current traces recorded from each cell. ( c ) Summary bar graph of TWIK-1 shRNA (TW1 shRNA), TWIK-1 rescue (TW1 insens WT) or TWIK-1 pore mutant (TW1 insens G119E) rescue currents plotted at −150 mV and +50 mV. Number on each bar indicates n for each condition. All values are mean±s.e.m. ( d ) Reversal potential ( V rev) of astrocytes in the TW1 shRNA-transfected and TW1 insens WT-transfected or TW1 insens G119E-transfected cells. Number on each bar indicates n for each condition. All values are mean±s.e.m. P -values were obtained with Student’s t -test. * P <0.05. Full size image TWIK-1 associates with TREK-1 in heterologous systems Based on the observation that TWIK-1 is functional in astrocytes, but not in COS-7 cells ( Supplementary Fig. 1b ), we hypothesized that functional expression of TWIK-1 may require certain factors expressed in astrocytes but not in COS-7 cells. To identify potential interacting partners for mouse TWIK-1, we performed conventional yeast two-hybrid (Y2H) and membrane Y2H screening using cytosolic N- and C termini and full-length TWIK-1 as bait. Among the positive clones that were isolated from three independent screens, we identified mouse TREK-1 as a binding partner protein of TWIK-1. We next confirmed the interaction between these two channels by using the full-length cDNAs of mouse TWIK-1 and mouse TREK-1. We found that TWIK-1 and TREK-1 formed a positive yeast colony in membrane Y2H under the non-permissive condition of the absence of threonine, leucine and histidine in yeast media (TLH−), while the empty vector did not ( Fig. 2a ). 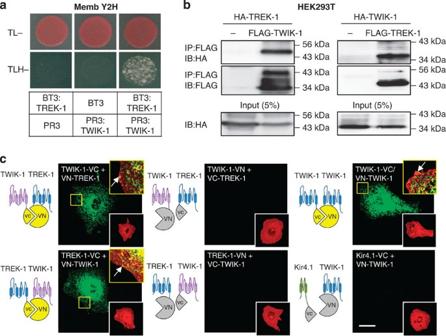Figure 2: TWIK-1 associates with TREK-1 in heterologous systems. (a) Identification of the TREK-1 as a direct binding partner of TWIK-1 in the novel split-ubiquitin yeast two-hybrid screen. (b) Co-immunoprecipitation assay in HEK293T cells. HA-TREK-1 and FLAG-TWIK-1 or HA-TWIK-1 and FLAG-TREK-1 were transfected into HEK293T cells and cell lysates were then immunoprecipitated using anti-HA antibody. The immunoprecipitates were examined by western blotting using anti-FLAG antibody. Input represented 5% of cell lysates used in the Co-IP assay. (c) Schematic diagram depicting the BiFC assay. VN and VC are the N-terminal and C-terminal fragments of the Venus, respectively. Intense Venus signals (green colour) are examined for dimerization. TWIK-1-VC strongly interacts with VN-TREK-1; TREK-1-VC also interacts with VN-TWIK-1. In the opposite orientation (TREK-1-VN and VC-TWIK-1 or TWIK-1-VN and VC-TREK-1), Venus signals were not detected. TWIK-1 homodimer is used as a positive control, and Kir4.1 and TWIK-1 heterodimer is used as a negative control. The fluorescent signals of BiFC were detected at the plasma membrane of the cells as indicated by the yellow colour (arrow, inset magnified image). Scale bar, 20 μm. Figure 2: TWIK-1 associates with TREK-1 in heterologous systems. ( a ) Identification of the TREK-1 as a direct binding partner of TWIK-1 in the novel split-ubiquitin yeast two-hybrid screen. ( b ) Co-immunoprecipitation assay in HEK293T cells. HA-TREK-1 and FLAG-TWIK-1 or HA-TWIK-1 and FLAG-TREK-1 were transfected into HEK293T cells and cell lysates were then immunoprecipitated using anti-HA antibody. The immunoprecipitates were examined by western blotting using anti-FLAG antibody. Input represented 5% of cell lysates used in the Co-IP assay. ( c ) Schematic diagram depicting the BiFC assay. VN and VC are the N-terminal and C-terminal fragments of the Venus, respectively. Intense Venus signals (green colour) are examined for dimerization. TWIK-1-VC strongly interacts with VN-TREK-1; TREK-1-VC also interacts with VN-TWIK-1. In the opposite orientation (TREK-1-VN and VC-TWIK-1 or TWIK-1-VN and VC-TREK-1), Venus signals were not detected. TWIK-1 homodimer is used as a positive control, and Kir4.1 and TWIK-1 heterodimer is used as a negative control. The fluorescent signals of BiFC were detected at the plasma membrane of the cells as indicated by the yellow colour (arrow, inset magnified image). Scale bar, 20 μm. Full size image To examine the interaction between these two proteins in a mammalian system, we constructed expression vectors for FLAG-tagged TWIK-1 (FLAG-TWIK-1) and haemagglutinin (HA)-tagged TREK-1 (HA-TREK-1) and co-expressed them in HEK293T cells. We then performed co-immunoprecipitation (Co-IP) on cell lysates with an anti-FLAG antibody and blotted with an anti-HA antibody. The results showed that HA-TREK-1 was strongly associated with FLAG-TWIK-1 ( Fig. 2b , left panel), an interaction that was confirmed by the reverse combination of HA-TWIK-1 and FLAG-TREK-1 expression vectors ( Fig. 2b , right panel). We then examined the interaction between TWIK-1 and TREK-1 at the single-cell level to verify the subcellular location of this interaction. To do this, we used the bimolecular fluorescence complementation (BiFC) technique [23] , which allows visualization of two independent proteins in close spatial proximity (a minimal distance of 7 nm (ref. 24 )). We constructed variants of TWIK-1 and TREK-1, whose N- and C terminus were fused with one complementary half of split Venus fluorescent protein, either the N-terminal half (VN) or the C-terminal half (VC), and then both were transfected into COS-7 cells ( Fig. 2c ). When the split Venus halves were on complementary positions in each subunit (TWIK-1-VC+VN-TREK-1 or TREK-1-VC+VN-TWIK-1), strong fluorescence was detected ( Fig. 2c , left panel). The BiFC fluorescent signals were detected at the plasma membrane of the cells, shown by the yellow colour (arrow, inset image in Fig. 2c ). However, with the split Venus halves in the opposite positions (TWIK-1-VN +VC-TREK-1 or TREK-1-VN+VC-TWIK-1), no fluorescence was detected ( Fig. 2c , middle panel). As a positive control, TWIK-1 homodimers [25] (TWIK-1-VC/VN-TWIK-1) showed the expected strong BiFC signals, but no complementation was observed between TWIK-1 and the inward rectifier Kir4.1 K + channel ( Fig. 2c , right panel). Further, when TWIK-1 or TREK-1 was expressed with only one half of split Venus, no fluorescence was detected ( Supplementary Fig. 2a ).These results strongly suggest that an association between TWIK-1 and TREK-1 occurs in live mammalian cells. TWIK-1 associates with TREK-1 in native astrocytes To determine whether such interactions between TWIK-1 and TREK-1 do indeed occur in astrocytes, we first examined the expression of K2P isoforms in these cells. Using real-time PCR, we found that TWIK-1 and TREK-1 are the predominant K2P isoforms of cultured astrocytes ( Supplementary Fig. 2b ). Immunocytochemical double labelling of TWIK-1 and TREK-1 proteins showed a strong co-localization in these cells ( Fig. 3a , Pearson’s correlation coefficient: 0.81±0.04, n =10). The specificity of antibodies against TWIK-1 ( Supplementary Fig. 2c ) and TREK-1 (ref. 20 ) was extensively documented. Co-IP experiments also demonstrated a strong association between native TWIK-1 and TREK-1 in astrocytes ( Fig. 3b ). 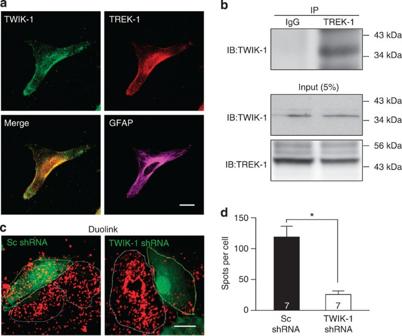Figure 3: TWIK-1 associates with TREK-1 in native astrocytes. (a) TWIK-1 co-localization with TREK-1 in astrocytes. Astrocytes were fixed and stained using specific antibodies for TWIK-1 and TREK-1. Co-localization was determined by merging individual panels. Scale bar, 20 μm. (b) Co-immunoprecipitation assay in astrocytes. Whole-cell lysates were immunoprecipitated using anti-TREK-1 antibody and then blotted using anti-TWIK-1 antibody. (c) Duolink PLA assay. Intense PLA signals were detected in Sc shRNA transfected astrocytes, but not in TWIK-1 shRNA transfected astrocytes. Scale bar, 20 μm. (d) The PLA signals were counted with Duolink Image Tool software and the average number of spots per cell is presented in the graph. Number on each bar indicatesnfor each condition. All values are mean±s.e.m.P-values were obtained with Student’st-test. *P<0.05. Figure 3: TWIK-1 associates with TREK-1 in native astrocytes. ( a ) TWIK-1 co-localization with TREK-1 in astrocytes. Astrocytes were fixed and stained using specific antibodies for TWIK-1 and TREK-1. Co-localization was determined by merging individual panels. Scale bar, 20 μm. ( b ) Co-immunoprecipitation assay in astrocytes. Whole-cell lysates were immunoprecipitated using anti-TREK-1 antibody and then blotted using anti-TWIK-1 antibody. ( c ) Duolink PLA assay. Intense PLA signals were detected in Sc shRNA transfected astrocytes, but not in TWIK-1 shRNA transfected astrocytes. Scale bar, 20 μm. ( d ) The PLA signals were counted with Duolink Image Tool software and the average number of spots per cell is presented in the graph. Number on each bar indicates n for each condition. All values are mean±s.e.m. P -values were obtained with Student’s t -test. * P <0.05. Full size image We found that this association was further supported by a Duolink proximity ligation assay ( Fig. 3c ). Duolink PLA labelling critically depends on close proximity (<40 nm) between interaction partners [26] . A strong PLA signal from TWIK-1 and TREK-1 was observed in astrocytes expressing Sc shRNA, but not in astrocytes expressing TWIK-1 shRNA ( Fig. 3c ). Quantification of the PLA signals under these conditions is shown in Fig. 3d . As a negative control, the Duolink PLA was performed in a mouse fibroblast cell line, NIH3T3, where little K2P is expressed. There was no positive PLA signal in these cells compared with native astrocytes ( Supplementary Fig. 2d ). Taking all findings together, we conclude that TWIK-1 and TREK-1 associate both in native astrocytes and in heterologous expression systems. TWIK-1/TREK-1 heterodimer requires a disulphide bridge Based on observations that TWIK-1 homodimerizes via a disulphide bridge [25] , [27] , a cysteine residue is located in the first extracellular loop of TREK-1 ( Fig. 4a ), and this cysteine residue is highly conserved in TWIK-1 and TREK-1 of several different species ( Supplementary Fig. 3a ), we considered the possibility that TWIK-1/TREK-1 heterodimer formation may be mediated by such a disulphide bridge. To examine this possibility, we constructed cysteine-to-serine [25] mutants of TWIK-1 (TWIK-1 C69S) and TREK-1 (TREK-1 C93S) and assessed their ability to interact. Our Co-IP analysis revealed a dramatic reduction in the association of each CS mutant with their wild-type binding partners ( Fig. 4b,c ). As a positive control, we confirmed that the disulphide bond is important for TWIK-1 homodimer formation ( Supplementary Fig. 3b ). However, TREK-1 homodimers did not require the disulphide bond ( Supplementary Fig. 3c ), a finding similar to that previously reported for TWIK-2 (ref. 28 ) and TASK-2 (ref. 29 ). 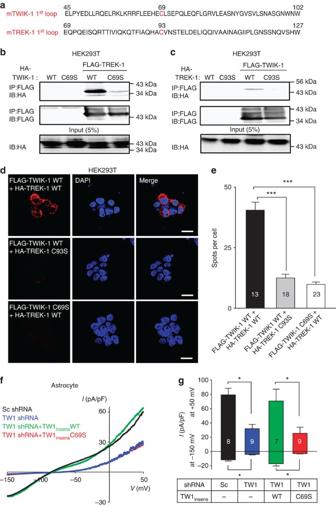Figure 4: TWIK-1 and TREK-1 heterodimer formation requires a disulphide bridge. (a) Comparison of first loop sequence in mouse TWIK-1 and mouse TREK-1. The cysteine residue is well conserved in two kinds of K2P channels. (b) Co-immunoprecipitation assays were performed on lysates of HEK293T cells co-expressing FLAG-TREK-1 and HA-TWIK-1 WT or C69S mutant. (c) Co-immunoprecipitation assays were performed on lysates of HEK293T cells co-expressing FLAG-TWIK-1 and HA-TREK-1 WT or C93S mutant. (d) Duolink PLA assay. Intense PLA signals were detected in only FLAG-WT-TWIK-1- and HA-WT-TREK-1-transfected HEK293T cells, but not in CS mutant-transfected HEK293T cells. Scale bar, 20 μm. (e) The PLA signals were counted with Duolink Image Tool software and the average number of spots per cell is presented in the graph. Number on each bar indicatesnfor each condition. All values are mean±s.e.m.P-values were obtained with Student’st-test. (f) Representative traces from Sc shRNA-transfected, TWIK-1 shRNA-transfected, TWIK-1 shRNA-insensitive form-transfected, or TWIK-1 shRNA-insensitive C69S transfected astrocytes. (g) Summary bar graph of Sc shRNA, TWIK-1 shRNA, TWIK-1 rescue or TWIK-1 C69S rescue currents plotted at −150 mV and +50 mV. Number on each bar indicatesnfor each condition. All values are mean±s.e.m.P-values were obtained with Student’st-test. *P<0.05, ***P<0.001. Figure 4: TWIK-1 and TREK-1 heterodimer formation requires a disulphide bridge. ( a ) Comparison of first loop sequence in mouse TWIK-1 and mouse TREK-1. The cysteine residue is well conserved in two kinds of K2P channels. ( b ) Co-immunoprecipitation assays were performed on lysates of HEK293T cells co-expressing FLAG-TREK-1 and HA-TWIK-1 WT or C69S mutant. ( c ) Co-immunoprecipitation assays were performed on lysates of HEK293T cells co-expressing FLAG-TWIK-1 and HA-TREK-1 WT or C93S mutant. ( d ) Duolink PLA assay. Intense PLA signals were detected in only FLAG-WT-TWIK-1- and HA-WT-TREK-1-transfected HEK293T cells, but not in CS mutant-transfected HEK293T cells. Scale bar, 20 μm. ( e ) The PLA signals were counted with Duolink Image Tool software and the average number of spots per cell is presented in the graph. Number on each bar indicates n for each condition. All values are mean±s.e.m. P -values were obtained with Student’s t -test. ( f ) Representative traces from Sc shRNA-transfected, TWIK-1 shRNA-transfected, TWIK-1 shRNA-insensitive form-transfected, or TWIK-1 shRNA-insensitive C69S transfected astrocytes. ( g ) Summary bar graph of Sc shRNA, TWIK-1 shRNA, TWIK-1 rescue or TWIK-1 C69S rescue currents plotted at −150 mV and +50 mV. Number on each bar indicates n for each condition. All values are mean±s.e.m. P -values were obtained with Student’s t -test. * P <0.05, *** P <0.001. Full size image To determine whether the CS mutation had any effect on the association within cells, we performed the Duolink PLA in HEK293T cells co-expressing FLAG-TWIK-1 and HA-TREK-1. Confocal images showed a strong PLA signal in HEK293T cells co-expressing wild-type TWIK-1 and TREK-1, but not for CS mutants of TWIK-1 or TREK-1 ( Fig. 4d,e ). In addition, we tested the effect of cystamine, an inhibitor of protein disulphide isomerase, on heterodimer formation in native astrocytes using Co-IP. Consistent with our prediction, cystamine treatment markedly reduced the association between TWIK-1 and TREK-1 in astrocytes ( Supplementary Fig. 3j ). To investigate the role of the disulphide bridge on TWIK-1 channel function, we measured I – V relationships in astrocytes transfected with both TWIK-1 shRNA and a shRNA-insensitive CS mutant of TWIK-1 (TWIK-1 insens C69S). We found that the TWIK-1 insens C69S could not rescue the effect of TWIK-1 shRNA in astrocytes, which was in striking contrast to that observed for wild-type TWIK-1 ( Fig. 4f,g ). In addition, cystamine treatment significantly reduced the background conductance of these cells ( Supplementary Fig. 3h,i ). These results suggest that the disulphide bridge between the two cysteine residues located in the first extracellular loop of each channel is critical for the formation of TWIK-1/TREK-1 heterodimers. Interdependence of TREK-1 and TWIK-1 for cell surface expression TWIK-1/TREK-1 heterodimer formation may be a requirement for cell surface expression of both proteins. To test for this possible interdependence, we first examined the influence of TREK-1 on cell surface expression of TWIK-1. When FLAG-TWIK-1 alone was transfected into COS-7 cells, FLAG-TWIK-1 failed to co-localize with DsRed-Mem ( Fig. 5a , top panel). However, in the presence of HA-TREK-1, co-localization of TWIK-1 and DsRed-Mem was increased substantially ( Fig. 5a,b ). Furthermore, a luminescence-based cell surface assay in COS-7 cells ( Fig. 5c ) and a surface biotinylation assay in HEK293T cells ( Fig. 5d ) both indicated that surface expression of TWIK-1 was markedly increased in the presence of TREK-1. Finally, co-expression of wild-type TWIK-1 and TREK-1 in COS-7 cells had a linear-like I – V relationship ( Supplementary Fig. 4d ), whereas cells expressing TWIK-1 or TREK-1 alone, showed insignificant currents or outwardly rectifying currents ( Supplementary Fig. 4a–c ). 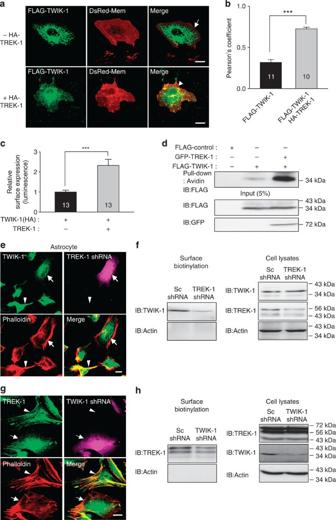Figure 5: TWIK-1 and TREK-1 are interdependently required for cell surface expression in astrocytes. (a) Plasma membrane localization of TWIK-1 in COS-7 cells. COS-7 cells were transfected with DsRed-Mem vector and FLAG-TWIK-1 in the absence (arrow) or presence (arrowhead) of HA-TREK-1 and were labelled with anti-FLAG antibody. Scale bar, 20 μm. (b) Pearson’s correlation coefficient denoting covariance of fluorescence signals was calculated using Nikon software. The Pearson’s correlation coefficient for TWIK-1 and DsRed-Mem in the presence of TREK-1 was significantly greater than values obtained from COS-7 cells in the absence of TREK-1. Number on each bar indicatesnfor each condition. All values are mean±s.e.m.P-values were obtained with Student’st-test. (c) Quantification of TWIK-1(HA) cell surface expression in the absence and presence of additional TREK-1 using anti-HA antibody. TWIK-1 cell surface expression is normalized to the average at TWIK-1-only expressing condition. Number on each bar indicatesnfor each condition. All values are mean±s.e.m.P-values were obtained with Student’st-test. (d) Cell surface biotinylation assay in HEK293T cells. When HEK293T cells were transiently transfected with GFP-TREK-1 and FLAG-TWIK-1, cell surface expression of TWIK-1 is dramatically increased. (e) Confocal immunofluorescence staining of TWIK-1 in TREK-1 shRNA transfected astrocytes. Fixed cells also stained with Alexa Fluo 647-labelled phalloidin for F-actin staining. Scale bar, 20 μm. (f) Cell surface biotinylation assay in TREK-1 shRNA-transfected astrocytes. (g) Confocal immunofluorescence staining of TREK-1 in TWIK-1 shRNA transfected astrocytes. Scale bar, 20 μm. (h) Cell surface biotinylation assay in TWIK-1 shRNA-transfected astrocytes. ***P<0.001. Figure 5: TWIK-1 and TREK-1 are interdependently required for cell surface expression in astrocytes. ( a ) Plasma membrane localization of TWIK-1 in COS-7 cells. COS-7 cells were transfected with DsRed-Mem vector and FLAG-TWIK-1 in the absence (arrow) or presence (arrowhead) of HA-TREK-1 and were labelled with anti-FLAG antibody. Scale bar, 20 μm. ( b ) Pearson’s correlation coefficient denoting covariance of fluorescence signals was calculated using Nikon software. The Pearson’s correlation coefficient for TWIK-1 and DsRed-Mem in the presence of TREK-1 was significantly greater than values obtained from COS-7 cells in the absence of TREK-1. Number on each bar indicates n for each condition. All values are mean±s.e.m. P -values were obtained with Student’s t -test. ( c ) Quantification of TWIK-1(HA) cell surface expression in the absence and presence of additional TREK-1 using anti-HA antibody. TWIK-1 cell surface expression is normalized to the average at TWIK-1-only expressing condition. Number on each bar indicates n for each condition. All values are mean±s.e.m. P -values were obtained with Student’s t -test. ( d ) Cell surface biotinylation assay in HEK293T cells. When HEK293T cells were transiently transfected with GFP-TREK-1 and FLAG-TWIK-1, cell surface expression of TWIK-1 is dramatically increased. ( e ) Confocal immunofluorescence staining of TWIK-1 in TREK-1 shRNA transfected astrocytes. Fixed cells also stained with Alexa Fluo 647-labelled phalloidin for F-actin staining. Scale bar, 20 μm. ( f ) Cell surface biotinylation assay in TREK-1 shRNA-transfected astrocytes. ( g ) Confocal immunofluorescence staining of TREK-1 in TWIK-1 shRNA transfected astrocytes. Scale bar, 20 μm. ( h ) Cell surface biotinylation assay in TWIK-1 shRNA-transfected astrocytes. *** P <0.001. Full size image We next used shRNA knockdown to examine the effect of TREK-1 depletion on cell surface expression of endogenous TWIK-1 in cultured astrocytes. The specificity of the TREK-1 shRNA has been documented previously [20] . Treatment with TREK-1 shRNA caused a dramatic reduction in cell surface expression of the endogenous TWIK-1 channel proteins, measured by surface biotinylation, in comparison to control Sc shRNA treatment, without affecting the total TWIK-1 protein levels ( Fig. 5f ). TREK-1 shRNA treatment also caused a loss of co-localization between TWIK-1 and phalloidin, a toxin that specifically labels F-actin [30] , which is known to be mainly located just beneath the plasma membrane in many cell lines and to co-localize with membrane proteins [31] , [32] , [33] . TWIK-1 was not co-localized with phalloidin in shRNA-treated cells ( Fig. 5e , arrow), whereas TWIK-1 co-localized with phalloidin in neighbouring non-transfected cells ( Fig. 5e , arrowhead). This suggests that TWIK-1 channel trafficking is affected by TREK-1 depletion. The reverse condition was also tested by examining the surface expression of TREK-1 while over-expressing TWIK-1 shRNA. We found that TWIK-1 shRNA caused a similar significant reduction in the cell surface expression of TREK-1, assessed with immunocytochemistry ( Fig. 5g ) and surface biotinylation ( Fig. 5h ). These data indicate that proper cell surface expression of both TWIK-1 and TREK-1 requires the presence of both binding partners. TWIK-1/TREK-1 is the major K2P channel in astrocytes In addition to forming heterodimers with TREK-1, TWIK-1 can also form homodimers via disulphide bridges ( Supplementary Fig. 3b ). However, most of these homodimers are not found at the cell surface ( Fig. 5a,b ). TREK-1 can also exist as a homodimer, without a disulphide bridge ( Supplementary Fig. 3c ), although for cell surface expression, this homodimer does require a disulphide bridge ( Supplementary Fig. 3f,g ). To determine the proportion of these channels that form TWIK-1/TREK-1 heterodimers, we compared the effect of knocking down TWIK-1 or TREK-1 alone with the effect of knocking down both proteins together. Treatment with TWIK-1 shRNA, TREK-1 shRNA and both shRNAs all significantly reduced both inward and outward currents in cultured astrocytes ( Fig. 6a–d ). To estimate the contribution of homodimers and heterodimers, we first subtracted currents measured after knockdown of TWIK-1 or TREK-1 from currents measured after double knockdown and then normalized to the currents measured after treatment of Sc shRNA at +50 mV or −150 mV ( Fig. 6e,f ). Assuming that each TWIK-1 shRNA or TREK-1 shRNA eliminates both homodimers and heterodimers, we deduced that the contribution of TWIK-1/TREK-1 heterodimers is >80%, with the remaining contribution coming mostly from TREK-1 homodimers, rather than TWIK-1 homodimers ( Fig. 6e,f ). 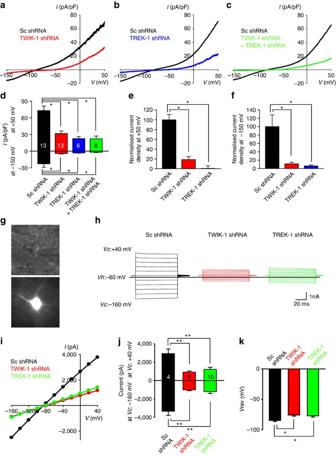Figure 6: Astrocytes express mostly the TWIK-1/TREK-1 heterodimer and it is this channel that regulates passive conductance. (a–c) Representative whole-cellI–Vcurves in astrocytes over-expressing Sc shRNA (black), TWIK-1 shRNA (red), TREK-1 shRNA (blue), or TWIK-1 and TREK-1 shRNAs (green). (d) Pooled data for whole-cell current amplitudes in TWIK-1 knockdown, TREK-1 knockdown or TWIK-1 and TREK-1 double knockdown astrocytes. Number on each bar indicatesnfor each condition. All values are mean±s.e.m. (e,f) Normalized current density. Data are mean±s.e.m. (g) DIC (upper) and fluorescence (lower) image of hippocampal astrocyte infected with mCherry-TREK-1 shRNA lentivirus in the CA1 striatum radiatum. Scale bar, 20 μM. (h) The whole-cell currents from hippocampal astrocytes infected with Sc (left) or TWIK-1 (middle) or TREK-1 (right) shRNA. Command voltage pulse protocol: voltages were stepped from −160 mV to +40 mV in increments of 20 mV from a holding potential of −60 mV. Dotted line indicates 0 pA. (i) The current–voltage relationship (I–V) from −160 mV to +40 mV. (j) The bar graph of current at −160 mV and +40 mV. Data are mean±s.e.m.P-values were obtained with Student’st-test. **P<0.01. Numbers of tested slices from at least two independent mice are indicated on each bar. (k) The bar graph representing reversal potential of respective conditions. Data are mean±s.e.m.P-values were obtained with Student’st-test. *P<0.05, **P<0.01. Figure 6: Astrocytes express mostly the TWIK-1/TREK-1 heterodimer and it is this channel that regulates passive conductance. ( a – c ) Representative whole-cell I – V curves in astrocytes over-expressing Sc shRNA (black), TWIK-1 shRNA (red), TREK-1 shRNA (blue), or TWIK-1 and TREK-1 shRNAs (green). ( d ) Pooled data for whole-cell current amplitudes in TWIK-1 knockdown, TREK-1 knockdown or TWIK-1 and TREK-1 double knockdown astrocytes. Number on each bar indicates n for each condition. All values are mean±s.e.m. ( e , f ) Normalized current density. Data are mean±s.e.m. ( g ) DIC (upper) and fluorescence (lower) image of hippocampal astrocyte infected with mCherry-TREK-1 shRNA lentivirus in the CA1 striatum radiatum. Scale bar, 20 μM. ( h ) The whole-cell currents from hippocampal astrocytes infected with Sc (left) or TWIK-1 (middle) or TREK-1 (right) shRNA. Command voltage pulse protocol: voltages were stepped from −160 mV to +40 mV in increments of 20 mV from a holding potential of −60 mV. Dotted line indicates 0 pA. ( i ) The current–voltage relationship ( I – V ) from −160 mV to +40 mV. ( j ) The bar graph of current at −160 mV and +40 mV. Data are mean±s.e.m. P -values were obtained with Student’s t -test. ** P <0.01. Numbers of tested slices from at least two independent mice are indicated on each bar. ( k ) The bar graph representing reversal potential of respective conditions. Data are mean±s.e.m. P -values were obtained with Student’s t -test. * P <0.05, ** P <0.01. Full size image TWIK-1/TREK-1 is a major contributor to passive conductance A recent report suggested that TWIK-1 and TREK-1 might independently contribute to the passive conductance of rat hippocampal astrocytes [21] . Thus, we tested whether TWIK-1/TREK-1 heterodimers contribute to this passive conductance. We directly measured the effects of knocking down TWIK-1 or TREK-1 in vivo by introducing TWIK-1 shRNA or TREK-1 shRNA into mice via lentivirus. Passive conductance of astrocytes was then measured in hippocampal slices prepared from injected mice ( Fig. 6g ). Compared with the control Sc shRNA, both TWIK-1 and TREK-1 shRNA markedly reduced astrocytic passive conductance ( Fig. 6h ). The I – V relationship showed that both outward and inward currents were dramatically reduced by each shRNA ( Fig. 6i,j ) and the reversal potential was shifted from −83 to about −77 mV ( Fig. 6k ). These findings strongly suggest that TWIK-1/TREK-1 heterodimers have a linear-like I – V relationship and are the major contributors to astrocytic passive conductance in vivo . The apparent difference in the shape of I – V relationships measured in cultured astrocytes (complex shape, for example, Fig. 6a ) and astrocytes in hippocampal slices (linear shape, for example, Fig. 6i ) is most likely due to inadequate spatial control of membrane potential resulting from the high leakage conductance of the astrocytes in slices [21] . To visualize and compare the astrocytic passive conductance mediated by the TWIK-1/TREK-1 heterodimer, TWIK-1 or TREK-1-mediated currents were obtained by isolating each shRNA-sensitive current in brain slices ( Fig. 7a ) and cultured astrocytes ( Fig. 7b ). TWIK-1- and TREK-1-mediated currents were similar in magnitude and shape in both cases, indicating a mutual dependency and the existence of the heterodimer. More importantly, these currents showed a similar linear-shaped I – V relationship. In comparison, heterologously expressed TWIK-1 and TREK-1 in COS-7 cells had a linear-like I – V relationship, although the current density was much lower compared with that in astrocytes ( Fig. 7c ). The linearity of the I – V relationship appears to be correlated with the degree of channel density as the order of linearity follows the order of channel density. These results reveal the shape of the I – V relationship of TWIK-1/TREK-1 heterodimer to be linear. 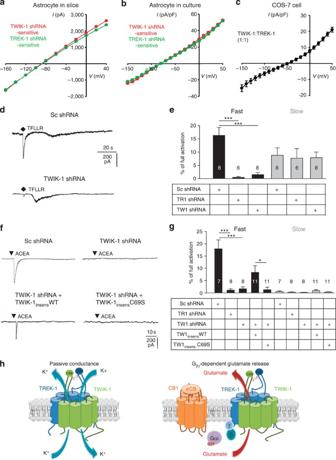Figure 7: TWIK-1/TREK-1 heterodimer releases glutamate upon CB1 activation in astrocytes. (a–c) AverageI–Vcurves for TWIK-1 or TREK-1 shRNA-sensitive currents in brain slices, cultured astrocytes and COS-7 cells expressing both TWIK-1 and TREK-1. (d) Representative traces for TFLLR-induced fast and slow glutamate release from astrocytes expressing Sc shRNA (upper panel) and TWIK-1 shRNA (lower panel). The diamonds indicate pressure application of TFLLR (100 ms, 0.1 s). (e) Summary bar graph for % of full activation of results from astrocytes expressing Sc shRNA, TREK-1 shRNA and TWIK-1 shRNA. All values are mean±s.e.m.P-values were obtained with Student’st-test. (f) Representative traces for ACEA-induced fast glutamate release from cultured astrocytes expressing Sc shRNA, TWIK-1 shRNA, TWIK-1 plus TWIK-1 shRNA-insensitive form (rescue), and TWIK-1 shRNA plus TWIK-1 shRNA-insensitive form C93S mutant (rescue control). (g) Summary bar graph for % of full activation of results from astrocytes expressing TWIK-1 plus TWIK-1 shRNA-insensitive form (rescue) and TWIK-1 shRNA plus TWIK-1 shRNA-insensitive form C93S mutant (rescue control). All values are mean±s.e.m.P-values were obtained with Student’st-test. (h) Schematic diagrams for passive conductance (left panel) and Gβγ-dependent glutamate release (right panel). *P<0.05, ***P<0.001. Figure 7: TWIK-1/TREK-1 heterodimer releases glutamate upon CB1 activation in astrocytes. ( a – c ) Average I – V curves for TWIK-1 or TREK-1 shRNA-sensitive currents in brain slices, cultured astrocytes and COS-7 cells expressing both TWIK-1 and TREK-1. ( d ) Representative traces for TFLLR-induced fast and slow glutamate release from astrocytes expressing Sc shRNA (upper panel) and TWIK-1 shRNA (lower panel). The diamonds indicate pressure application of TFLLR (100 ms, 0.1 s). ( e ) Summary bar graph for % of full activation of results from astrocytes expressing Sc shRNA, TREK-1 shRNA and TWIK-1 shRNA. All values are mean±s.e.m. P -values were obtained with Student’s t -test. ( f ) Representative traces for ACEA-induced fast glutamate release from cultured astrocytes expressing Sc shRNA, TWIK-1 shRNA, TWIK-1 plus TWIK-1 shRNA-insensitive form (rescue), and TWIK-1 shRNA plus TWIK-1 shRNA-insensitive form C93S mutant (rescue control). ( g ) Summary bar graph for % of full activation of results from astrocytes expressing TWIK-1 plus TWIK-1 shRNA-insensitive form (rescue) and TWIK-1 shRNA plus TWIK-1 shRNA-insensitive form C93S mutant (rescue control). All values are mean±s.e.m. P -values were obtained with Student’s t -test. ( h ) Schematic diagrams for passive conductance (left panel) and G βγ -dependent glutamate release (right panel). * P <0.05, *** P <0.001. Full size image TWIK-1/TREK-1 releases glutamate upon CB1 activation Astrocytes rapidly release glutamate via a TREK-1-containing K2P channel upon the activation of GPCRs such as protease-activated receptor-1 (PAR1) [20] . This glutamate release is initiated when the C terminus of the G γ subunit, GNG4, binds to the N terminus of TREK-1 to open the glutamate-permeable, TREK-1-containing K2P channel [20] . Of interest to note, is that data from Y2H screening using cytosolic N- and C termini of TWIK-1 showed that GNG4 is also bound to both cytosolic parts of this channel. We used Y2H and MBP pull-down assays to establish that TWIK-1 can directly bind to the G γ subunit ( Supplementary Fig. 5a,b ). In addition, to see whether G βγ can directly open glutamate-permeable channels, we constructed a concatenated TWIK-1/TREK-1 heterodimer and expressed this construct in COS-7 cells. We found that direct infusion of G βγ opened Cl − - and glutamate-permeable channels with an estimated permeability ratio of P glutamate / P Cl =0.27 ( Supplementary Fig. 7 ), according to the Goldman–Hodgkin–Katz equation. This permeability ratio is comparable to the ratio value of P glutamate / P Cl =0.27, as previously obtained from the G βγ -induced current in cultured astrocytes [20] . These results indicate that TWIK-1/TREK-1 heterodimer shows substantial permeability to glutamate upon G βγ binding. Next, to determine whether TWIK-1/TREK-1 heterodimers are responsible for fast glutamate release, we performed sniffer-patch recordings on astrocytes expressing Sc shRNA, TREK-1 shRNA or TWIK-1 shRNA. Sniffer patch is a highly sensitive bioassay for the detection of glutamate release [20] . We found that TWIK-1 shRNA almost completely and selectively eliminated the fast glutamate release elicited by the application of TFLLR, an agonist of PAR1, without affecting the slow component of glutamate release ( Fig. 7d,e ). Similar effects were observed with TREK-1 shRNA ( Fig. 7e ), as previously reported [20] . These results indicate that TWIK–1/TREK-1 heterodimers are also responsible for fast glutamate release in astrocytes. CB1 is a G αi -linked GPCR that is highly expressed in astrocytes. Activation of CB1 is known to release glutamate, though the mechanism of CB1-induced glutamate release has been controversial [34] , [35] , [36] , [37] . We wondered therefore whether CB1-induced glutamate release is due to TWIK-1/TREK-1 heterodimers. We found that application of the CB1 agonist, ACEA, induced fast glutamate release from astrocytes and this release was completely inhibited by either TWIK-1 shRNA or by TREK-1 shRNA ( Fig. 7f ). Co-expression of TWIK-1 insens WT with TWIK-1 shRNA fully rescued fast glutamate release, whereas the C69S mutant form of TWIK-1 insens (TWIK-1 insens C69S) failed to do so ( Fig. 7g ). These results indicate that TWIK-1/TREK-1 heterodimers are responsible for fast glutamate release induced by the activation of CB1 ( Fig. 7h ). The present study uncovers the mysterious function of TWIK-1 by identifying the long unknown channel responsible for the passive conductance of astrocytes. We provide strong evidence that TWIK-1 becomes a functional channel in astrocytes only after becoming a heterodimer with TREK-1, another member of the K2P family. This TWIK-1/TREK-1 heterodimer requires a disulphide bridge that is formed between two cysteine residues in the first extracellular loop of each channel. Furthermore, we demonstrate that TWIK-1/TREK-1 heterodimers are not only the major contributors to the passive conductance of astrocytes, but are also involved in CB1-induced fast glutamate release from these cells. Although there have been previous clear indications of TWIK-1 expression in various tissues, such as kidney, lung and brain [3] , [38] , [39] , TWIK-1 has been thought to be a non-functional or silenced channel [7] , [40] , [41] . Our study demonstrates that TWIK-1 requires a partner subunit for proper cell surface expression. This new mechanism for functional expression of TWIK-1 is profoundly different from the previously suggested silencing mechanisms for TWIK-1 involving endocytosis or sumoylation [8] . Nevertheless, the TWIK-1/TREK-1 heterodimer appears to be actively regulated by endocytosis ( Supplementary Fig. 6a,b ), although not by sumoylation ( Supplementary Fig. 6c,d ). It is plausible that the diverse regulatory processes that are known to affect TREK-1 homomeric channels—including mechano-, lipid- and thermo-sensitivity, as well as modulation by GPCRs—could also affect the activity of TWIK-1/TREK-1 heterodimers. Further studies will be needed to fully understand the regulatory mechanisms of TWIK-1/TREK-1 heterodimers. The conserved cysteine in the first extracellular loop of TWIK-1 and TREK-1 is also found in several isotypes of K2P channels such as the TWIK, TREK, and TALK subfamilies. Thus, it is possible that heterodimers might be formed between diverse K2P isotypes. In fact, we found that TWIK-1 can also form heterodimers with TREK-2 or TRAAK via a disulphide bridge ( Supplementary Fig. 3d,e ). Although the disulphide bridge is critical for TWIK-1-mediated dimerization, for TWIK-1 homodimer ( Supplementary Fig. 3b ) and TWIK-1/TREK-1 heterodimer formation ( Fig. 4b,c ), for example, it may not be required for other types of K2P channels. Previous studies showed that a disulphide bridge is not required for the formation of TWIK-2 (ref. 28 ) or TASK-2 (ref. 29 ) homodimers. Our results also demonstrated that TREK-1 homodimers do not require a disulphide bridge ( Supplementary Fig. 3c ). Thus, other unidentified mechanisms must exist for dimerization of K2P channels. This idea is further supported by a previous report showing TASK-1/TASK-3 heterodimer formation in the absence of cysteine residues normally present in the first loop of each channel [42] , [43] . It was recently reported that TWIK-1 can assemble with TASK-1 or TASK-3, but not with TREK-1, in live Chinese Hamster Ovary cells using the fluorescence resonance energy transfer (FRET) technique, though no detailed molecular mechanism was provided [44] . In this report, TWIK-1 showed no positive FRET signal with TREK-1, which appears to be in direct contrast to our positive finding of a strong BiFC signal ( Fig. 2c ). However, after careful examination of the report, we see that the discrepancy arises from technical limitations of the FRET and BiFC techniques. Although these techniques are powerful tools that permit visualization of protein–protein interactions [45] , [46] , the distance between two fluorescent proteins within the constructs is the most important factor for achieving a positive signal [24] , [47] . Indeed, our BiFC experiments showed that some combination of constructs (TWIK-1-VC+VN-TREK-1 or TREK-1-VC+VN-TWIK-1) gave a strong fluorescence signal ( Fig. 2c , left panel), while others (TWIK-1-VN+VC-TREK-1 or TREK-1-VN+VC-TWIK-1) gave no signal at all ( Fig. 2c , middle panel). Therefore, a lack of FRET signal in one combination of constructs does not necessarily mean a lack of interaction between the two subunits [48] . Other combinations of TWIK-1 and TREK-1 for FRET imaging should be investigated to resolve this discrepancy. We have recently demonstrated a unique function of TREK-1-containing K2P channels in releasing glutamate from astrocytes upon binding of G βγ [20] . In the present study, we have extended this analysis by demonstrating that TWIK-1/TREK-1 heterodimers are the precise molecular entities responsible for the fast mode of glutamate release upon activation of G αi -coupled GPCRs (CB1 in particular) in astrocytes. In addition to G protein-coupled inwardly rectifying K + channels (GIRKs) [49] and the alpha subunits of some voltage-gated Ca 2+ channels [50] , this TWIK-1/TREK-1 heterodimer is the third known case of G βγ binding to ion channels. We demonstrate here that K + -permeable TWIK-1/TREK-1 heterodimer channels can change their ion selectivity to allow large molecules such as glutamate to permeate upon binding of G βγ . Although alteration of ion selectivity is a rare phenomenon, it has been previously reported in a few ion channels, such as TRPV1 (ref. 51 ) and P2X7 (ref. 52 ). Notably, some K2P channels have unusual pore domain sequences [53] . Unlike conventional K + channels that contain GYG motifs in their pore domains, TWIK-1 has GYG and GLG motifs in the first and second pore domains, whereas TREK-1 has GFG motifs in both pore domains [53] . The existence of such unconventional pore domains may contribute to the mechanism underlying pore dilation and raises the possibility that these channels are permeable to other ions, such as sodium or chloride. For example, TWIK-1 has been shown to be responsible for the abnormal sodium permeability of human heart during pathological hypokalaemia [6] . TREK-1 is also known to be permeable to sodium ions when the first 56 amino acids of the N-terminal domain are omitted by alternative translational initiation [54] . These data imply that the N terminus of TREK-1 is important for ion selectivity of this channel. In astrocytes, G βγ -induced currents are mediated by direct interaction of G βγ with the N terminus of TREK-1 and are carried by chloride ions and even by glutamate [20] . We show in this study that the concatenated TREK-1–TWIK-1 heterodimer can be permeable to chloride ions and glutamate upon G βγ application ( Supplementary Fig. 7a,b ). These data imply that the pore region of the TWIK-1/TREK-1 heterodimer is altered upon G βγ application. Therefore, both the unique pore domain sequence and its ability to bind to G βγ seem to induce a pore change in TWIK-1/TREK-1 heterodimers that allows permeation of large molecules such as glutamate. The precise nature and characteristics of the glutamate-permeable pore is unknown. It is possible that the K + selective pore is either the same or different from the glutamate-permeable pore. In TWIK-1 shRNA-expressing astrocytes, the pore mutant of TWIK-1, TWIK-1 insens G119E, failed to rescue the background conductance and reversal potential ( Fig. 1c–e ), indicating that the TWIK-1 pore is responsible for K + permeation. The CB1-induced fast glutamate release ( Supplementary Fig. 8 ) however was fully rescued, indicating that the TWIK-1 pore is not responsible for glutamate permeation. In contrast to that seen for the TWIK-1 pore, we have previously shown that the TREK-1 pore is responsible for both K + permeation and glutamate permeation [20] . Therefore, a more detailed analysis of the structural and conformational changes of TWIK-1/TREK-1 heterodimer will be required to clarify the nature of the pore and the mechanism of G βγ -induced glutamate release. Finally, we identified the TWIK-1/TREK-1 heterodimer as being the ion channel responsible for the passive conductance in hippocampal astrocytes. Although the TWIK-1/TREK-1 heterodimer is responsible for the majority of the passive conductance, there is still a residual conductance of some 30% that is unaccounted for by gene silencing of either TWIK-1 or TREK-1 shRNA, which suggests that other K + channels contribute. We tested whether Kir4.1 or TREK-2 was involved in the remaining passive conductance and found that passive conductance was slightly affected by Kir4.1 but not by TREK-2 ( Supplementary Fig. 9c–e ). Thus, it remains unclear which type of K + channel may be involved in the residual passive conductance after knockdown of the TWIK-1/TREK-1 heterodimer. It is also possible that a partial gene silencing of TWIK-1 or TREK-1 might be responsible for the residual conductance, although each shRNA displayed >90% knockdown efficiency in a heterologous expression system. Future studies with TWIK-1 or TREK-1 null mice will be helpful to determine the precise contribution of heterodimers and homodimers to the passive conductance in astrocytes. In conclusion, our new insights into how TWIK-1 forms functional channels in astrocytes suggest that K2P channels may exist as many diverse combinations of isotypes that are linked by disulphide bridges. Furthermore, TWIK-1/TREK-1 heterodimers mediate diverse functions ranging from the passive conduction of K + in resting astrocytes to the fast release of glutamate in stimulated astrocytes. The new concepts and tools developed in our study should prove useful for further improvements in understanding the functional roles of brain astrocytes in various physiological and pathological conditions. Chemicals N -5 Z ,8 Z ,11 Z ,14 Z -eicosatetraenamide (ACEA) was purchased from Tocris, USA. TFLLR was synthesized by Peptron, Korea. Pluronic acid (F-127) and Fura-2 AM were purchased form Molecular Probes, USA. Cystamine dihydrochloride was purchased from Sigma. Purified G βγ protein was purchased from Calbiochem (catalogue no. 371768). Plasmids and shRNA cDNAs encoding for full-length mouse TREK-1 (GenBank accession no. NM_010607 ), mouse TWIK-1 (NM_008430), mouse Kir4.1 (GenBank accession no. NM_001039484 ), mouse TREK-2 (GenBank accession no. NM_029911 ) and mouse SENP1 (BC023129) were obtained by using an RT–PCR-based gateway cloning method (Invitrogen). Dynamin 2 WT and K44A constructs were obtained from Dr Jang (Seoul National University). CS mutants of TREK-1 and TWIK-1 were also generated using full-length cDNAs as templates via the EZchange site-directed mutagenesis kit (Enzynomics). All constructs were cloned into several vectors, including pDEST-FLAG-C, pDEST-HA-C and pDEST-IRES2-GFP by gateway cloning. The target region of shRNA as follows: mouse TWIK-1: 5′-GCATCATCTACTCTGTCATCG-3′; mouse TREK-1: 5′-GCGTGGAGATCTACGACAAGT-3′; mouse TREK-2: 5′-GCAGTCAGAAGAACACAATCG-3′; mouse Kir4.1: 5′-GCTACAAGCTTCTGCTCTTCT-3′. TWIK-1 shRNA-insensitive form (5′-GCATAATATATAGCGTGG-3′), TWIK-1 pore mutant (G119E), TWIK-1 C69S mutant and TREK-1 C93S were obtained by performing oligonucleotide-directed mutagenesis using the EZchange site-directed mutagenesis kit. For construction of concatenated TREK-1 and TWIK-1, TREK-1 and TWIK-1 were re-cloned into pDONR207 P1P5R and pDONR207 P5P2 vectors respectively via two independent BP-reactions (Invitrogen), and then performing a MultiSite Gateway LR recombination reaction (Invitrogen) according to the manufacturer’s guidelines, combining pDONR207-TREK-1, pDONR207-TWIK-1 and pDEST-IRES2-GFP. Primary cortical astrocytes Primary cortical astrocytes were prepared from 1–3-day-old male and female C57BL/6 mouse pubs [55] . The cerebral cortex was dissected free of adherent meninges, minced and dissociated into a single-cell suspension by trituration. All experimental procedures described were performed in accordance with the institutional guidelines of the Korea Institute of Science and Technology (KIST, Seoul, Korea). Cells were grown in Dulbecco’s modified Eagle’s medium (DMEM, Invitrogen) supplemented with 25 mM glucose, 10% heat-inactivated horse serum, 10% heat-inactivated fetal bovine serum, 2 mM glutamine and 100 units per ml of penicillin–streptomycin. Cultures were maintained at 37 °C in a humidified 5% CO 2 incubator. On the third day of culture, cells were vigorously washed with repeated pipetting and the media was replaced to remove debris and other floating cell types. On the next day (fourth day of culture), cells were replated onto glass coverslips (1 × 10 4 per coverslip) coated with 0.1 mg ml −1 Poly D -Lysine (PDL), and during this procedure cultured astrocytes were transfected with various cDNAs and shRNAs by electroporation. Human embryonic kidney (HEK) 293T cells and COS-7 cells HEK293T cells and COS-7 cells were purchased from the Korean Cell Line Bank (Seoul National University) and cultured in DMEM (Invitrogen) supplemented with 10% fetal bovine serum (Invitrogen), 100 units per ml penicillin–streptomycin at 37 °C in a humidified atmosphere of 95% air and 5% CO 2 . Transfection of expression vectors was performed with Lipofectamine 2000 (Invitrogen), according to the manufacturer’s protocol. One day prior to performing sniffer-patch experiments, HEK293T cells were transfected with 1:10 ratio of green fluorescence protein (pEGFP-N1) and pCINeo-GluR1-L497Y (5 μg per 60 mm dish) or 1:3 red fluorescence protein (pDsRed) and pCINeo-GluR1-L497Y using Effectene (Qiagen). CNQX (5 μM) was always supplemented in the medium to block AMPA receptor-mediated cytotoxicity. Transfection of astrocytes On the fourth day of culture, when astrocytes were replated onto glass coverslips, primary cultured astrocytes were electroporetically transfected with various cDNAs or shRNAs with an optimized voltage protocol (1,100 V, 20 pulse width, 2 pulses) using the Microporator (Invitrogen). Cell number for each transfection was 2 × 10 6 . The transfected cells were loaded onto coverslips and cultured for at least 36 h. On the day of sniffer patch, transfected astrocytes were mixed with HEK293T cells expressing GluR1-L497Y. The following cDNAs and shRNAs were used: 5 μg pSicoR-TWIK-1 shRNA or pSicoR-TREK-1 shRNA for blocking mouse TWIK-1 or TREK-1 expression, respectively; pSicoR-TWIK-1 shRNA and pIRES2-GFP-TWIK-1 insens (shRNA-insensitive form) for rescue experiments; pSicoR-TWIK-1 shRNA and pSicoR-TREK-1 shRNA for blocking both mouse TWIK-1 and TREK-1 expression; pSicoR-TWIK-1 shRNA and pIRES2-GFP-TWIK-1 insense G119E for confirming pore mutants, and pSicoR-TWIK-1 shRNA and pIRES2-GFP-TWIK-1 insens C69S for demonstrating the importance of the cysteine bridge in the TWIK-1/TREK-1 heterodimer. Split-ubiquitin membrane-based yeast two-hybrid assay Polypeptides that interact with the bait protein bring together the C-terminal fragment (Cub) and a modified N-terminal fragment (NubG, isoleucine 13 replaced by glycine) of ubiquitin, allowing ubiquitin-specific proteases (UBPs) to liberate PLV (protein A, LexA and VP16) from Cub, which then is free to enter the nucleus and activate transcription of the lacZ and His3. The TREK-1 was ligated into pBT3 encoding for the Cub, LexA and VP16, and the TWIK-1 was cloned into pPR3 encoding for the NubG. To assess the protein–protein interaction between TREK-1 and TWIK-1, both pBT3/TREK-1 and pPR3/ TWIK-1 were co-transformed into the yeast strain NMY51. NMY51 is unable to synthesize histidine. However, interaction between TWIK-1 and TREK-1 enables the yeast to make the His3 enzyme, thereby permitting histidine biosynthesis and growth on His minimal medium. Co-immunoprecipitation and immunoblotting For co-immunoprecipitation, whole-cell lysates were mixed overnight at 4 °C with 1 μg ml −1 anti-HA (F-7; Santa Cruz Biotechnology) or anti-TREK-1 (H-75; Santa Cruz Biotechnology) antibodies in lysis buffer (50 mM Tris–HCl, pH 7.4, 150 mM NaCl, 5 mM EDTA, 1 mM PMSF and 1% NP-40) containing a protease-inhibitor cocktail (Roche). Immune complexes were incubated by binding to mixed protein A/G PLUS-Agarose (Santa Cruz Biotechnology) for 1 h and then washed four times with lysis buffer. For immunoblotting, protein samples were separated by SDS–PAGE using 10% gels. The separated proteins were transferred to polyvinylidene fluoride membranes. The blots were incubated overnight at 4 °C with anti-HA antibody (Roche Applied Science; 3F10, 1:1,000), anti-FLAG antibody (Sigma; F1804, 1:1,000) or anti-TWIK-1 antibody (Alomone Labs; # APC-110, 1:500). Blots were then washed and incubated with horseradish peroxidase-conjugated goat anti-mouse, goat anti-rat or anti-rabbit IgG, followed by washing and detection of immunoreactivity with enhanced chemiluminescence (Amersham Biosciences). Full gel scans of all western blot in this paper can be found in Supplementary Fig. 10 . Cell surface biotinylation and surface expression assay For surface biotinylation, the cell surface proteins of FLAG-TWIK-1-transfected HEK293T cells or TREK-1 shRNA or TWIK-1 shRNA-infected astrocytes were incubated at 4 °C and washed three times with PBS. Cell surface-expressed proteins were then biotinylated in PBS containing Sulfo-NHS-SS-Biotin (Pierce, Rockford, IL, USA) for 30 min. After biotinylation, cells were washed with quenching buffer (100 mM glycine in PBS) to remove excess biotin and then washed three times with PBS. The cells were then lysed and incubated with high capacity NeutrAvidin-Agarose Resin (Thermo Scientific). After three washes with lysis buffer, bound proteins are eluted by the SDS sample buffer and subjected to western blot analysis. For surface expression analysis, a haemagglutinin (HA) tag (YPYDVPDYA) was inserted at the second loop end of TWIK-1 as previously reported with TREK-1(HA) [56] . HA-inserted TWIK-1 (TWIK-1(HA)) and GFP-TREK-1 were transfected into HEK293T cells. After 24 h, transfected cells were fixed in 4% paraformaldehyde for 20 min at 4 °C and incubated in PBS containing 5% BSA for 30 min at 4 °C to block non-specific binding of primary antibodies. Cells were then incubated with 1 μg ml −1 rat monoclonal anti-HA antibody (3F10, Roche Applied Science) in PBS containing 2% FBS for 1 h at 4 °C, washed three times with ice-cold PBS and then incubated with HRP-coupled goat anti-rat antibody (Jackson Immunoresearch Labs) in PBS containing 2% FBS for 1 h at 4 °C. The cells were gently washed three times with ice-cold PBS and then lysed for 30 min on ice in lysis buffer. Individual cells were placed into 50 μl SuperSignal ELISA Femto solution (Pierce) and after an equilibration period of 30 s, chemiluminescence was quantified with a M200 pro luminometer (Tecan). Each construct surface expression of cells was analysed in one experiment and at least three experiments were performed. Immunocytochemistry The specificities of TREK-1 antibody (Alomone Labs; #APC-047, 1:100) and TWIK-1 antibody (Santa Cruz Biotechnology; sc-11483, 1:50) were assessed with immunocytochemistry in cultured astrocytes in combination with TREK-1 shRNA or TWIK-1 shRNA. Primary cultured astrocytes were transfected with TREK-1 shRNA or TWIK-1 shRNA and grown on coverslips for an additional 48 h. The COS-7 cells growing on coverslips were co-transfected with FLAG or HA-fused channel vectors using Lipofectamine 2000 (Invitrogen). The cells were fixed in 4% paraformaldehyde for 20 min at room temperature, then permeabilised with PBS with 0.5% NP-40 for 5 min. Non-specific binding was prevented with 1 h incubation in 2% Donkey Serum (GeneTex). Cells were incubated overnight, at 4 °C, with the anti-TREK-1 (Alomone Labs, #APC-047, 1:200), anti-TWIK-1 (Santa Cruz Biotechnology; sc-11483, 1:100), anti-GFAP (Millipore; AB5541, 1:500), anti-HA antibody (Roche Applied Science; 3F10, 1:100) and anti-FLAG antibody (Sigma; F1804, 1:100). After washing, DyLight 488-, 549- or 649-conjugated secondary antibody (Jackson Labs, 1:400) was added and incubated for 1 h at room temperature. The cells were washed and mounted, and then observed under a Nikon A1 confocal microscope. When needed, the plasma membrane localization vector, DsRed-Mem (Clontech Laboratories) was co-transfected with the FLAG or HA-fused channel vectors. To quantify co-localization of the merged images, >10 cells were randomly analysed. Co-localization of multiple sets of optical images was quantified with Nikon A1 confocal microscope software to obtain Pearson’s correlation coefficients. BiFC assay For BiFC, TWIK-1, TREK-1 and Kir4.1 were cloned into bimolecular fluorescence complement (pBiFC)-VN173 and pBiFC-VC155 vectors. COS-7 cells were co-transfected with cloned BiFC vectors in all possible pairwise combinations and then transfected with DsRed-Mem for the detection of plasma membrane. The next day, these cells fixed with 4% paraformaldehyde for 20 min at room temperature and mounted with Dako Fluorescence Mounting Medium. Venus fluorescence signals were observed by confocal microscopy. Duolink proximity ligation assay Interaction was detected by Duolink proximity ligation assay kit (Olink Bioscience, Uppsala, Sweden: PLA Probe anti-Rabbit MINUS; PLA Probe anti-Goat PLUS; Detection Kit 563). The PLA probe anti-Rabbit MINUS binds to the TREK-1 antibody (Alomone Labs), whereas the PLA probe anti-Goat PLUS binds to the TWIK-1 antibody (Santa Cruz Biotechnology). If the distance between both proteins is <40 nm, a signal with DuoLink PLA is generated, thus indicating an interaction between both proteins [25] . After pre-incubation with a blocking agent for 1 h, the fixed astrocytes were incubated overnight with the primary antibodies to TREK-1 (Alomone Labs, 1:200) and TWIK-1 (Santa Cruz Biotechnology, 1:100). Duolink PLA probes detecting rabbit or goat antibodies were diluted in the blocking agent to a concentration of 1:5 and applied to the slides, followed by incubation for 2 h in a pre-heated humidity chamber at 37 °C. Unbound PLA probes were removed by washing. For hybridization of the two Duolink PLA probes, Duolink Hybridization stock (dilution 1:5) was used. The slides were incubated in a pre-heated humidity chamber for 15 min at 37 °C, and were then incubated in the ligation solution consisting of Duolink Ligation stock (1:5) and Duolink Ligase (1:40) for 90 min at 37 °C. Detection of the amplified probe was performed with the Duolink detection kit. Duolink Detection stock was diluted at 1:5 and applied for 1 h at 37 °C. Final washing steps were carried out in saline sodium citrate buffer. Electrophysiological recording in cultured astrocytes Cultured astrocytes at days 3–4 were transiently transfected by electroporation. After transfection cells were plated onto coverslips and maintained in DMEM supplemented with 10% fetal bovine serum and 10% horse serum for at least 48 h before electrophysiology experiments. Transfected astrocytes were identified by fluorescence using an Olympus IX71 inverted microscope equipped with an Andor iXon3 digital camera. Recording pipettes were fabricated from borosilicate glass capillaries (World Precision Instruments) using a P-97 Flaming/Brown micropipette puller (Sutter Instruments). The pipettes had an open-tip resistance of 3–4 MΩ when filled with a pipette solution containing (in mM): 150 KCl, 1 CaCl 2 , 1 MgCl 2 , 5 EGTA and 10 HEPES (pH 7.2 was adjusted with KOH). Standard bath solution contained (in mM): 150 NaCl, 3 KCl, 2 CaCl 2 , 1 MgCl 2 , 10 HEPES, 5.5 D-glucose and 20 sucrose (pH 7.4 was adjusted with NaOH). The mean membrane resistance of hippocampal astrocytes in culture is 7.45±0.76 mega ohms (mean±s.e.m. ), and the series resistance was <15 mega ohms, which we monitored throughout experiments. Whole-cell membrane currents were amplified by the Axopatch 200A. Currents were elicited by 1-s ramps descending from +50 mV to −150 mV (from a holding potential of −70 mV). Data acquisition was controlled by pCLAMP 10.2 software (Molecular Devices). The Digidata 1322A interface was used to convert digital–analogue signals between amplifier and computer. Data were sampled at 5 kHz and filtered at 2 kHz. Cell membrane capacitance was measured by using the ‘membrane test’ protocol built into pClampex. All experiments were conducted at a room temperature of 20–22 °C. Electrophysiological recording in COS-7 cells Current–voltage ( I – V ) curves were recorded from COS-7 cells expressing TWIK-1, TREK-1 or concatenated TREK-1-TWIK-1-IRES2-GFP. I – V curves were established by applying 1000-ms-duration voltage ramps from +100 to −100 mV. For measuring G βγ -induced chloride currents, recording electodes (4–7 MΩ) were filled with (mM): 145 NMDG-Cl, 0.5 CaCl 2 , 10 HEPES, 4 Mg-ATP, 0.3 Na 3 -GTP, 10 BAPTA and 6.09 nM G βγ (pH adjusted to 7.3 with CsOH). Bath solution was shifted from HEPES buffer (in mM: 150 NaCl, 10 HEPES, 3 KCl, 2 CaCl 2 , 2 MgCl 2 and 5.5 glucose, pH 7.3) to NMDG buffer (in mM: 145 NMDG-Cl, 10 HEPES, 3 KCl, 2 CaCl 2 , 2 MgCl 2 and 5.5 glucose, pH 7.3). For measuring G βγ -induced glutamate current, recording electrodes (4–7 MΩ) were filled with (mM): 145 NMDG-glutamate, 0.5 CaCl 2 , 10 HEPES, 4 Mg-ATP, 0.3 Na 3 -GTP, 10 BAPTA and 6.09 nM G βγ (pH adjusted to 7.3 with CsOH). Whole-cell membrane currents were amplified using the Axopatch 200A patch clamp system. Currents were elicited by 1-s ramps descending from +50 mV to −150 mV (from a holding potential of −70 mV). Data acquisition was controlled by pCLAMP 10.2 software (Molecular Devices). A Digidata 1322A interface was used to convert digital–analogue signals between amplifier and computer. Data were sampled at 5 kHz and filtered at 2 kHz. Cell membrane capacitance was measured using the ‘membrane test’ protocol built into pClampex. All experiments were conducted at a room temperature of 20–22 °C. Construction and delivery of shRNA–lentiviral vectors For gene silencing in vivo , the validated mouse shRNA sequences for TWIK-1, TREK-1, TREK-2 and Kir4.1 were cloned into the lentiviral pSicoR vector using XhoI/XbaI sites [57] , and high-titer lentiviral vectors were produced by KIST virus facility (Korea). Briefly, the lentiviral vectors were produced by co-transfecting each pSicoR vector with the ViraPower lentiviral packaging mix (Invitrogen) in the 293FT packaging cell line. The supernatant was collected and concentrated by ultracentrifugation. For astrocyte-specific shRNA delivery, lentiviral vectors were always produced at subneutral pH ( ⩽ pH 7.0) [58] and injected into hippocampal CA1 region (AP: 0.17, ML: 0.17, DV: 0.19) of 7–8-week-old wild-type C57BL/6 mice. Electrophysiological recording in hippocampal astrocytes The virus-infected mouse brain slices (350 μm) containing hippocampus were acutely prepared using a vibrating blade microtome (Leica VT1000 S) [55] . Prepared slices were left to recover for at least 1 h before recording in oxygenated (95% O 2 and 5% CO 2 ) artificial cerebrospinal fluid (ACSF; in mM, 130 NaCl, 24 NaHCO 3 , 3.5 KCl, 1.25 NaH 2 PO 4 , 1 CaCl 2 , 3 MgCl 2 and 10 glucose, pH 7.4; at room temperature). Individual hippocampal slices were transferred to the recording chamber, which was constantly perfused with ACSF recording solution composed of (in mM) 130 NaCl, 24 NaHCO 3 , 3.5 KCl, 1.25 NaH 2 PO 4 , 1.5 CaCl 2 , 1.5 MgCl 2 and 10 glucose saturated with 95% O 2 –5% CO 2 , at pH 7.4. Acute brain slices were co-loaded with SR-101 (Sigma; 1 μM) dye to identify the location of astrocytes in the CA1 region. Patch pipettes had a resistance of 5–7 MΩ when filled with pipette solution composed of (in mM): 140 KCl, 10 HEPES, 5 EGTA, 2 Mg-ATP, 0.2 NaGTP, adjusted to pH 7.4 with KOH. Whole-cell patch recordings were performed in hippocampal astrocytes with a voltage-clamp configuration using an Axopatch 200 A (Axon Instruments, Union City, CA, USA). The mean membrane resistance of hippocampal astrocytes in slices is 4±1.2 mega ohms (mean±s.e.m.). And the series resistance was <30 mega ohms, which we monitored throughout the experiment. The calculated and measured junction potential is −2.6 mV and −2.5 mV, respectively. Sniffer patch Sniffer patch was composed of Fura-2 imaging for Ca 2+ from astrocytes and current recordings from HEK293T cells expressing GluR1-L497Y. To release glutamate from astrocytes, PAR1 and CB1 were activated by pressure application of TFLLR peptide and ACEA, respectively. On the day of experiments, cultured mouse astrocytes (HEK293T cells added) were incubated with 5 mM Fura-2 AM (mixed with 5 ml of 20% pluronic acid; Invitrogen) for 40 min, washed at room temperature and subsequently transferred to the microscope stage for imaging. External solution contained (in mM): 150 NaCl, 10 HEPES, 3 KCl, 2 CaCl 2 , 2 MgCl 2 and 5.5 glucose (pH adjusted to pH 7.3 and osmolarity adjusted to 325 mOsmol kg −1 ). Intensity images of 510 nm wavelength were taken at 340 nm and 380 nm excitation wavelengths with an iXon EMCCD camera (Andor). Two resulting images were used for ratio calculations in Imaging Workbench version 6.2 (Indec Systems). GluR1L497Y-mediated current recordings were acquired from HEK293T cells under voltage clamp (Vh of −70 mV) using a Multiclamp 700B amplifier and pClamp 9.2 software (Molecular Devices). Recording electrodes (4–7 MU) were filled with (mM): 110 Cs-gluconate, 30 CsCl, 0.5 CaCl 2 , 10 HEPES, 4 Mg-ATP, 0.3 Na 3 -GTP and 10 BAPTA (pH adjusted to 7.3 with CsOH and osmolarity adjusted to 290–310 mOsm kg −1 ). To test whether glutamate release involved TWIK-1, we used pSicoR-TWIK-1-shRNA to gene-silence TWIK-1 expression and pIRES2-GFP-TWIK-1-insensitive form for rescue experiments. Yeast two-hybrid assay The N- or C termini of TWIK-1 were ligated into pGBKT7 encoding for the GAL4 DNA binding domain (BD) and GNG4 was cloned into pGADT7 encoding for the activation domain (AD). BD/TWIK-1-N or -C and AD/GNG4 were co-transformed into the yeast strain AH109, in order to assess the protein–protein interaction of GNG4 with TWIK-1-N or TWIK-1-C. AH109 is unable to synthesize histidine. However, both TWIK-1-N and -C with GNG4 enable the yeast to make the His3 enzyme, thereby permitting histidine biosynthesis and growth on His minimal medium. MBP pull-down assay For MBP pull-down assays, MBP–GNG4 fusion protein was transformed into the E. coli strain BL21 using the pMGWA expression vector. According to the manufacturer’s protocol, MBP–GNG4 protein was purified (SpinClean; Mbiotech). GFP-tagged TWIK-1-N or TWIK-1-C were transfected into HEK293T cells and extracted after 24 h. The cell lysates were incubated with 3 μg of purified MBP–GNG4 and immobilized on MBP Bind agarose resin (Elpis Biotech Inc., Korea) for 1 h at 4 °C. After three washes with lysis buffer, bound proteins are eluted by SDS sample buffer and subjected to western blot analysis. Real-time PCR Total RNA was isolated from mouse cultured astrocytes using an RNA purification Kit (GeneAll, Korea) according to the manufacturer’s instructions. cDNA was synthesized from 1 μg total RNA and reverse transcription was performed using a SuperScript VILO cDNA Synthesis Kit (Invitrogen) according to the manufacturer’s instructions. Real-time PCR was performed using a TaqMan Gene Expression assay (Invitrogen). Primer sets for TWIK-1, TREK-1, TREK-2, TRAAK, TASK-1, TASK-2, TASK-3, TALK-1 and TRESK-2 were purchased from IDT (PrimeTime qPCR assay). GAPDH was used as a housekeeping gene. Primer sequence information is listed in Supplementary Table S1 . Experiments were repeated a minimum of three times. The 2 ΔΔ C t method was used to calculate fold changes in gene expression [59] . Data analysis and statistical analysis Off‐line analysis was carried out using Clampfit and SigmaPlot software. Co-localization analysis of multiple sets of optical images was quantified using Nikon A1 confocal microscope software. Pearson’s correlation coefficients ( r ) were calculated from the co-localization signals at the edge region of cells, from 10 different cells, with the same software, and at least 10 different edge regions per one cell were analysed. The r values are between 0 and 1. A value of 1 means that perfect co-localization occurs, while a value of 0 means that no co-localization is seen. Numerical data are presented as mean±s.e.m. The significance of data for comparison was assessed by Student’s two-tailed unpaired t -test and significance levels were given as: * P <0.05, ** P <0.01 and *** P <0.001. How to cite this article: Hwang, E. M. et al . A disulphide-linked heterodimer of TWIK-1 and TREK-1 mediates passive conductance in astrocytes. Nat. Commun. 5:3227 doi: 10.1038/ncomms4227 (2014).